Manganese hexacyanomanganate open framework as a high-capacity positive electrode material for sodium-ion batteries Potential applications of sodium-ion batteries in grid-scale energy storage, portable electronics and electric vehicles have revitalized research interest in these batteries. However, the performance of sodium-ion electrode materials has not been competitive with that of lithium-ion electrode materials. Here we present sodium manganese hexacyanomanganate (Na 2 Mn II [Mn II (CN) 6 ]), an open-framework crystal structure material, as a viable positive electrode for sodium-ion batteries. We demonstrate a high discharge capacity of 209 mAh g −1 at C/5 (40 mA g −1 ) and excellent capacity retention at high rates in a propylene carbonate electrolyte. We provide chemical and structural evidence for the unprecedented storage of 50% more sodium cations than previously thought possible during electrochemical cycling. These results represent a step forward in the development of sodium-ion batteries. Lithium-ion batteries (LIBs) dominate the energy storage market for portable electronics and play a crucial role in the deployment of electric vehicles because of their superior power and energy densities [1] . Technological developments and economies of scale from widespread use in electric vehicles are expected to reduce their cost substantially in the near future, but concerns regarding the future availability of lithium resources are rising [2] . In addition, their application in grid-scale electrochemical energy storage is attractive because of their high performance and ease of deployment, but currently they are still too expensive [3] . As a result, sodium (Na)-ion batteries (NIBs), which replace lithium with abundant and inexpensive Na, have received a great deal of attention recently [4] . Similarities in manufacturing process between NIBs and LIBs may significantly accelerate their technological advance [4] , [5] . Nevertheless, several scientific challenges still need to be resolved before the performance of NIBs becomes competitive with that of LIBs. In particular, the higher negative redox potential of Na compared with that of Li results in lower cell voltages and consequently lower energy densities [4] . Moreover, the larger size of Na + relative to Li + (1.02 versus 0.69 Å) causes slower solid-state diffusion in the active materials and leads to lower energy efficiencies when the batteries are rapidly charged or discharged [6] . High-capacity electrode materials with fast solid-state kinetics are therefore required in order to compensate for these intrinsic limitations of NIBs. In the past, researchers have explored the possibility of adapting positive electrode materials of LIBs, including Na super ionic conductor structures [7] , layered oxides [5] , [8] , tunnel-structured oxides [9] and fluorophosphates [10] , for Na + intercalation. However, close-packed, oxide-ion arrays connected by first-row transition metal elements do not have enough interstitial space in the structure for rapid Na + diffusion [11] . This is why layered-oxide structures, such as Na x [Fe 1/2 Mn 1/2 ]O 2 (ref. 5 ), are promising candidates from a specific capacity standpoint (190 mAh g −1 ) but suffer from poor Na + transport kinetics (32% capacity retention at 4C; ref. 11 ). On the other hand, Na super ionic conductor and fluorophosphates exhibit better rate performance (93% capacity retention at 4C), but their bulky three-dimensional network structures limit their specific capacity to 130 mAh g −1 (refs 7 , 10 ). The discovery of a positive electrode material that combines high-specific Na + storage capacity with high rate capability has remained an open challenge. Prussian Blue analogues (PBAs) have been explored for many different applications because of their ease of synthesis and intriguing electrochemical and magnetic properties [11] , [12] , [13] , [14] , [15] . Their general chemical formula is A x P[R(CN) 6 ] 1− y □ y ˙ n H 2 O (A: mobile cations; P: nitrogen-coordinated transition metal ion; R: carbon-coordinated transition metal ion; □: [R(CN) 6 ] vacancy; 0≤ x ≤2; 0≤ y <1). PBAs typically possess the well-known, face-centered cubic crystal structure with the Fm-3m space group, in which transition metal ions are linked together through cyanide (CN) ligands ( Fig. 1a ). Each unit cell consists of eight subunit cells and therefore contains eight interstitial sites that can host various ions, such as Li + , Na + , K + , NH 4 + , Rb + , alkaline earth divalent ions and zeolitic water [16] , [17] . The open-framework nature of the cubic structure, which contains open <100> channels (3.2 Å in diameter) and interstitial sites (4.6 Å in diameter) in the case of Prussian Blue [18] , enables rapid solid-state diffusion of a wide variety of ions. The electrochemical properties of PBAs can be ascribed to the redox behaviour of the transition metal ions in either the P or R sites. 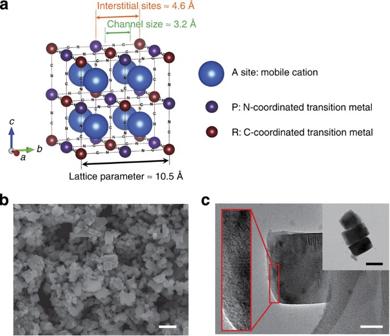Figure 1: Schematic illustration of cubic PBAs and morphology of as-synthesized MnHCMn. (a) The general structure of open-framework PBAs consists of a face-centered cubic phase. Owing to the lengthy CN bonds, subunit cells contain large interstitial sites. (b,c) SEM (b) (scale bar, 500 nm) and TEM (c) (white scale bar, 30 nm; black scale bar of insert image, 100 nm) images show the morphology of MnHCMn, which is composed of cubic particles ~100 nm in size. We use monovalent A + ions as an example: Figure 1: Schematic illustration of cubic PBAs and morphology of as-synthesized MnHCMn. ( a ) The general structure of open-framework PBAs consists of a face-centered cubic phase. Owing to the lengthy CN bonds, subunit cells contain large interstitial sites. ( b , c ) SEM ( b ) (scale bar, 500 nm) and TEM ( c ) (white scale bar, 30 nm; black scale bar of insert image, 100 nm) images show the morphology of MnHCMn, which is composed of cubic particles ~100 nm in size. Full size image Depending on the type of transition metal ions, their oxidation states, the concentration and type of cations in the interstitial sites, and the concentration of hexacyanometallate vacancies, structural distortions triggered by changes in the CN bonding of the original cubic structure to monoclinic, rhombohedral or orthorhombic may occur [19] , [20] , [21] , [22] . In the case of a general, vacancy-free PBA, the theoretical capacity owing to storage of monovalent cations results from the occupation of each of the eight empty interstitial sites with A + ions ( Fig. 1a ) and is 171 mAh g −1 in the case of Prussian Blue (FeHCFe). Recently, we and others have utilized PBAs as battery electrodes with excellent cycle life and rate performance in both aqueous and organic electrolytes for NIBs [11] , [12] , [13] , [23] , [24] , [25] , [26] , [27] , [28] , [29] . In this Article, we introduce manganese hexacyanomanganate (Na 2 Mn II [Mn II (CN) 6 ]=MnHCMn) as a viable positive electrode material for NIBs. The as-synthesized MnHCMn has a monoclinic crystal structure composed of nonlinear Mn–N≡C–Mn bonds ( Supplementary Figs 1 and 2 ) and contains eight large interstitial sites occupied by Na + ions. Our experiments demonstrate a surprisingly high-specific capacity of 209 mAh g −1 in organic electrolyte, which is substantially more than the 172 mAh g −1 that would be expected for vacancy-free MnHCMn if each interstitial site were occupied by a single Na + ion. Through a thorough chemical and structural analysis, we explain the origin of the improved capacity and describe the mechanism underlying this phenomenon. Electrochemical properties of Na manganese hexacyanomanganate MnHCMn was synthesized by a solution precipitation method described in the Methods section below. The precise composition of the as-synthesized material was determined by elemental analysis, inductively coupled plasma mass spectrometry (ICP-MS) and thermogravimetric analysis to be Na 1.96 Mn[Mn(CN) 6 ] 0.99 □ 0.01 ·2H 2 O ( Supplementary Fig. 3 ). The concentration of hexacyanometallate vacancies is extremely low compared with other PBAs, and this is achieved by using a large excess of Na + in solution during the synthesis [30] . The morphology and size of MnHCMn were confirmed by scanning electron microscopy and transmission electron microscopy (TEM) in Fig. 1b,c . The images show cubic particles with an average size of 100 nm. The TEM image indicates that the particles have lattice fringes with a single orientation, which makes them highly crystalline. Electrochemical performance of the material as positive electrode is shown in Fig. 2 . Galvanostatic voltage profiles in Fig. 2a clearly show the reversible specific capacity of MnHCMn. The discharge capacity at C/5 (40 mA g −1 ) reaches 209 mAh g −1 with a coulombic efficiency of 99.5%. The three plateaus in the voltage profile at ~1.8, 2.65 and 3.55 V versus Na 0 /Na + are ascribable to the redox reactions of Mn II –N≡C–Mn II/I , Mn II –N≡C–Mn III/II and Mn III/II –N≡C–Mn III , respectively, according to a study of standard potentials in metal hexacyanometallates [16] , [23] . Mn II –N≡C–Mn II/I and Mn II –N≡C–Mn III/II mean that the carbon-coordinated Mn atoms (R sites) in the structure are electrochemically active, while Mn III/II –N≡C–Mn III means that the nitrogen-coordinated Mn atoms (P sites) are. 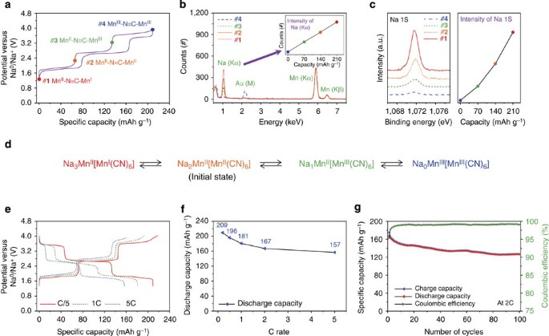Figure 2: Electrochemical properties and Na+ion concentration in MnHCMn. (a) Galvanostatic charge and discharge curves at C/5. The samples were prepared by initially discharging and then charging to the end points of each reaction plateau. The first discharge curve is reported inSupplementary Fig. 4. (b,c) EDS (b) and XPS (c) data show consistently increasing Na peak intensities as MnHCMn is reduced, which corresponds to the electrochemical insertion of Na+ions throughout the full voltage range of cycling. (d) The schematic illustrates the nominal compositions of MnHCMn at the end points of each Na+ion insertion reaction plateau. (e,f) Charge and discharge curves (e) and rate capability (f) as a function of different C rates are shown. (g) MnHCMn exhibits promising capacity retention over 100 cycles at 2C. Figure 2: Electrochemical properties and Na + ion concentration in MnHCMn. ( a ) Galvanostatic charge and discharge curves at C/5. The samples were prepared by initially discharging and then charging to the end points of each reaction plateau. The first discharge curve is reported in Supplementary Fig. 4 . ( b , c ) EDS ( b ) and XPS ( c ) data show consistently increasing Na peak intensities as MnHCMn is reduced, which corresponds to the electrochemical insertion of Na + ions throughout the full voltage range of cycling. ( d ) The schematic illustrates the nominal compositions of MnHCMn at the end points of each Na + ion insertion reaction plateau. ( e , f ) Charge and discharge curves ( e ) and rate capability ( f ) as a function of different C rates are shown. ( g ) MnHCMn exhibits promising capacity retention over 100 cycles at 2C. Full size image The electrochemical insertion of Na + ions in MnHCMn was confirmed by energy-dispersive X-ray spectroscopy (EDS) and X-ray photoelectron spectroscopy (XPS) spectra, as shown in Fig. 2b,c . Samples with four different states of charge (# 1 : Mn II –N≡C–Mn I ; # 2 : Mn II –N≡C–Mn II ; # 3: Mn II –N≡C–Mn III and # 4: Mn III –N≡C-Mn III ) were prepared by galvanostatic charge and discharge at C/5 ( Fig. 2a ). If we plot the normalized Na (Kα) peak intensities ( Fig. 2b ), we observe a linear correlation with the electrochemical specific capacity. The XPS Na 1 s peak intensities also increase as MnHCMn is discharged from # 4 to # 1 ( Fig. 2c left), thus confirming Na + insertion with electrode discharge. The XPS at the Mn 2p edge was also measured ( Supplementary Fig. 5 ), but the complexity of the chemical structure made the determination of the Mn valence state on each plateau inconclusive. Each of the three plateaus during galvanostatic cycling accounts for ~70 mAh g −1 , giving a total specific capacity of 209 mAh g −1 . Based on these results and on the known composition of the as-synthesized material, we are able to calculate the chemical formula for the four states of charge schematically shown in Fig. 2d . The electrochemical measurements give values of x =3.00, 2.04, 1.07 and 0.00 for Na x Mn[Mn(CN) 6 ] 0.99 □ 0.01 ·2H 2 O for the four redox states, which agrees well with the nominal chemical formula in Fig. 2d . When the C-rate increases to 1C and beyond, the capacity retention remains above 90 and 95% for the reactions at 2.65 and 1.8 V, respectively, as shown in Fig. 2e . The overall rate capability is excellent. We observe 75% capacity retention from C/5 to 5C ( Fig. 2f ), and most of the capacity decrease is at the 3.55 V plateau ( Fig. 2e ). This behaviour at 3.55 V is consistent with previous observations of low rate capacity and cycling stability of the nitrogen-coordinated Mn II/III redox couple in PBAs as a result of local charge redistribution and structural distortion [31] . The data in Fig. 2g illustrates promising cycle life, with 75% capacity retention after 100 cycles at 2C with high coulombic efficiency of 99.2% (see Supplementary Fig. 6 for additional cycling data at C/5). Structural phase transformations between oxidation states In order to understand the mechanism behind the unusually high capacity of MnHCMn, we used synchrotron X-ray diffraction (XRD) to study the structural characteristics of the material with cycling, as shown in Fig. 3 . 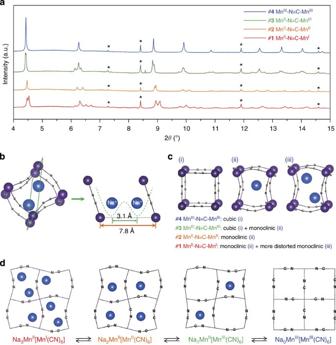Figure 3: Phase transitions and geometric considerations for two Na+ions within one subunit cell. (a) Synchrotron XRD patterns of MnHCMn at the end points of each reaction plateau (#1to #4inFig. 2a) within the initial cycle illustrate the different structures associated with each redox state. The orthorhombic phase (#3) includes peaks that resemble those of both cubic (#4) and monoclinic (#2) phases, and the fully reduced phase (#4) includes peaks that resemble those of both the monoclinic phase (#2) and a second more heavily distorted monoclinic phase. Asterisks (*) indicate the XRD peaks of the sodium chloride (NaCl) reference, which was used to calibrate peak positions across different samples. (b) In the fully discharged state, half of the subunit cells should contain two Na+ions. Na+ions are drawn along thecaxis towards the carbon-coordinated Mn, which leaves sufficient space within the structure for two ions. (c) Localized structural distortions in the initial cycle depend on the number of Na+ions within each subunit cell. (d) The schematic diagrams illustrate the changes in structure for MnHCMn during battery cycling. Figure 3a shows the XRD patterns of MnHCMn at the end points of each reaction plateau (samples # 1 to # 4 in Fig. 2a ) within the initial cycle. Asterisks (*) in Fig. 3a indicate the XRD peaks of the sodium chloride (NaCl) reference, which was used to calibrate peak positions across different samples. Structureless Le Bail fits of the XRD data were generated to identify the space groups and lattice parameters for MnHCMn in each oxidation state, as shown in Supplementary Fig. 7 . Figure 3: Phase transitions and geometric considerations for two Na + ions within one subunit cell. ( a ) Synchrotron XRD patterns of MnHCMn at the end points of each reaction plateau (# 1 to # 4 in Fig. 2a ) within the initial cycle illustrate the different structures associated with each redox state. The orthorhombic phase (# 3 ) includes peaks that resemble those of both cubic (# 4 ) and monoclinic (# 2 ) phases, and the fully reduced phase (# 4 ) includes peaks that resemble those of both the monoclinic phase (# 2 ) and a second more heavily distorted monoclinic phase. Asterisks (*) indicate the XRD peaks of the sodium chloride (NaCl) reference, which was used to calibrate peak positions across different samples. ( b ) In the fully discharged state, half of the subunit cells should contain two Na + ions. Na + ions are drawn along the c axis towards the carbon-coordinated Mn, which leaves sufficient space within the structure for two ions. ( c ) Localized structural distortions in the initial cycle depend on the number of Na + ions within each subunit cell. ( d ) The schematic diagrams illustrate the changes in structure for MnHCMn during battery cycling. Full size image The as-synthesized MnHCMn possesses a monoclinic phase with a space group of P2 1 / n and the following lattice parameters: a M =10.669 Å, b M =7.605 Å, c M =7.409 Å, α M = γ M =90 ° and β M =92.43 ° . These lattice parameters differ by <0.04% compared with those observed by Kareis et al. [32] in their study of Na-containing MnHCMn. A MnHCMn electrode that has been electrochemically reduced and oxidized back to the initial oxidation state (# 2 : Mn II –N≡C–Mn II ) possesses the same monoclinic space group and lattice parameters as the as-synthesized powder. The XRD data for fully oxidized Mn III –N≡C–Mn III (# 4 ) shows the typical perovskite cubic peaks corresponding to the Fm-3m space group and lattice parameters of a C = b C = c C =10.706 Å. Le Bail fitting of partially reduced Mn II –N≡C–Mn III (# 3 ) matches the orthorhombic space group P222 1 with lattice parameters of a O =10.688 Å, b O =7.724 Å, c O =7.477 Å. Fitting of the fully reduced Mn II –N≡C–Mn I (# 1 ) corresponds to the monoclinic space group P2 1 with lattice parameters of a M ′ =11.051 Å, b M ′ =7.525 Å, c M ′ =7.862 Å, α M ′ = γ M ′ =90 ° and β M ′ =108.84 ° , which is more distorted than the as-synthesized monoclinic phase (sample # 2 ). Although these four crystal structures seem to have distinct symmetries and lattice parameters within the initial cycle, the orthorhombic and monoclinic cells are equivalent to slightly distorted versions of the cubic cell if they are rotated by 45 ° around the a axis. The orthorhombic and monoclinic lattice parameters can be converted to their corresponding cubic lattice parameters: Mn II –N≡C–Mn I : a 1 =10.459 Å and b 1 = c 1 =10.905 Å; Mn II –N≡C–Mn II : a 2 =10.658 Å and b 2 = c 2 =10.616 Å; and Mn II –N≡C–Mn III : a 3 =10.688 Å and b 3 = c 3 =10.750 Å. Compared with the cubic Mn III –N≡C–Mn III , the unit cells expand or shrink only <3% throughout the range of electrochemical cycling ( Supplementary Table 1 ), which reflects the stable crystal structure of open-framework PBAs [12] , [33] . The overall volume expansion is 1.36%, which is the lowest value ever observed for NIBs [10] . The fully reduced Mn II –N≡C–Mn I , which has a molecular formula of Na 3 Mn II [Mn I (CN) 6 ], is scientifically intriguing because such a high Na-ion content has never been observed in PBAs before. In fact, this is only possible if four of the eight interstitial sites in each unit cell are occupied by not one but two Na + ions on average. Each subunit cell consists of four Mn 2+ and four [Mn(CN) 6 ] 4− in the as-synthesized state of Mn II –N≡C–Mn II . Na + ions are not stable at the octahedral centre of the subunit cell owing to attraction towards the more electronegative [Mn(CN) 6 ] 4− , which draws the Na + ions in the <111> directions towards the four tetrahedral sites in each subunit cell [20] . In the most discharged state, the stronger interaction between Na + and [Mn(CN) 6 ] 5− drives further displacement of Na + ions, which creates sufficient space for two Na + ions. Simple geometric calculations predict that there is space for a Na + –Na + distance of 3.1 Å, as shown in Fig. 3b . By comparison, the Li + –Li + distance in LiCoO 2 , a typical layered-oxide battery electrode material, is 2.81 Å. Moreover, the Na + –Na + distance in P2-type Na x [Fe 1/2 Mn 1/2 ]O 2 is 2.96 Å (ref. 5 ). Thus, the open-framework structure of MnHCMn has sufficient space for two Na + ions within a subunit cell in its fully discharged form. A conceptually straightforward way to visualize this ion storage mechanism is to assign each of the eight subunit cells its own local structure ( Fig. 3c ). An empty subunit cell is cubic, a subunit cell with one Na + ion is monoclinic, and a subunit cell with two Na + ions has a more heavily distorted monoclinic shape. Thus, the orthorhombic phase, which has Na + ions occupying half of the subunit cells, is composed of cubic and monoclinic subunit cells. A unit cell in Mn II –N≡C–Mn I (# 1 ) consists of four monoclinic subunit cells (occupied by a single Na + ion) and four more heavily distorted monoclinic subunit cells (occupied by two Na + ions; Fig. 3c ). Indeed, several XRD peaks (shown by arrows in Fig. 3a ) of Mn II –N≡C–Mn III (# 3 ) correspond to the superposition of peaks from both cubic (# 4 ) and monoclinic (# 2 ) MnHCMn. Likewise, some peaks of Mn II –N≡C–Mn I (# 1 ) correspond to those of the monoclinic Mn II –N≡C–Mn II (# 2 ) phase, as shown in Fig. 3a , while the remaining peaks match a more heavily distorted monoclinic phase owing to the presence of two Na + ions within one subunit cell. Despite all of these local structural distortions, the overall unit cell does not change much beyond minor distortions in the framework, as shown in the schematic illustrations shown in Fig. 3d . In the quest to replace Li-ion batteries in energy storage systems, scientists have looked for low-cost, earth-abundant and environmentally benign materials with high performance. MnHCMn, which has an open-framework crystal structure, can be synthesized by a simple co-precipitation method at room temperature that may minimize the processing costs during industrial production. The material is primarily composed of manganese, which is earth-abundant and non-toxic, and is therefore suitable for low-cost battery applications. The reversible capacity of 209 mAh g −1 at an average voltage of 2.65 V versus Na 0 /Na + makes the material promising as a positive electrode material for NIB applications. This high capacity has been achieved primarily because of the presence of three distinct Na + ion insertion steps during cycling. The open-framework structure enables structural integrity while accommodating multiple Na + ions, which leads to both fast kinetics and high capacity. Thus, we believe that MnHCMn represents a novel and scientifically intriguing material that can push forward the development of practical NIBs. Synthesis of MnHCMn Monoclinic Na manganese (II) hexacyanomanganate (II) MnHCMn was prepared by a co-precipitation method adapted from the literature [34] . An aqueous solution of Mn(NO 3 ) 2 ·4H 2 O (0.25 M) was added to an aqueous solution of NaCN (1.28 M) in the presence of an excess of NaCl (50:1 mol:mol) in a dark container within a N 2 -filled glovebox. The blue precipitate was centrifuged, washed twice with 30 ml of distilled H 2 O, twice with 30 ml of acetonitrile and then dried under vacuum for 24 h at room temperature. Materials characterization The compositions were determined by the standard microanalytical method for C, H and N elements and by ICP-MS for Na and Mn elements. High-resolution synchrotron powder XRD patterns were obtained with a wavelength of 0.413737 Å through the mail-in programme at beamline 11-BM at the Advanced Photon Source at Argonne National Laboratory. XRD patterns were indexed using the CRYSFIRE Powder Indexing System [35] . Le Bail fits for calculating space groups and crystal structures were prepared with General Structure Analysis System/Experiment Graphical User Interface (GSAS/EXPGUI) [36] , [37] . For elemental analysis, TEM (FEI Tecnai G 2 F20 X-Twin microscope, acceleration voltage 200 kV) equipped with an EDS spectrometer was used. To avoid the peak overlap of Na K α and Cu L α , a Au grid was used for clear determination of the Na concentration. The relative amounts of Na ions in each sample were determined by comparing the ratios of the integrated peak areas near 1 keV for Na and from 5.6–6.8 keV for Mn. The absolute ionic ratios were calibrated to the composition of as-synthesized MnHCMn using data from ICP-MS mentioned above. Typically, the EDS acquisition time was 300 s for all spectra, which allows for good signal-to-noise ratios. Electrochemical measurement To prepare electrodes, 80 wt.% active material of MnHCMn, 13 wt.% carbon black (Timcal Super P Li) and 7 wt.% polyvinylidene fluoride (Kynar HSV 900) were ground in an agate mortar in 1-methyl-2-pyrrolidone to form a slurry. Slurries of MnHCMn working electrodes were coated on carbon cloth current collectors (Fuel Cell Earth /Ballard AvCarb) with mass loadings of ~10 mg cm −2 . Afterwards, the electrodes were dried in vacuum at room temperature for 10 h. Electrochemical measurements were performed on flooded three-electrode cells. The cells contain a Ag/AgCl mesh as a pseudo-reference electrode and an activated carbon counter electrode. Each Ag/AgCl mesh pseudo-reference electrode was calibrated relative to the ferrocene (Fc + /Fc) redox couple ( Supplementary Fig. 8 ). This electrochemical setup guarantees an accurate measurement of the potential, excluding any contribution from the counter electrode. Two electrode, coin cell measurements using a Na metal-negative electrode show similar results ( Supplementary Fig. 9 ). Electrochemical characterizations were performed using a BioLogic VMP3 multi-channel battery tester at room temperature. How to cite this article: Lee, H.-W. et al. Manganese hexacyanomanganate open framework as a high-capacity positive electrode material for sodium-ion batteries. Nat. Commun. 5:5280 doi: 10.1038/ncomms6280 (2014).